AAA+ chaperones and acyldepsipeptides activate the ClpP protease via conformational control The Clp protease complex degrades a multitude of substrates, which are engaged by a AAA+ chaperone such as ClpX and subsequently digested by the dynamic, barrel-shaped ClpP protease. Acyldepsipeptides (ADEPs) are natural product-derived antibiotics that activate ClpP for chaperone-independent protein digestion. Here we show that both protein and small-molecule activators of ClpP allosterically control the ClpP barrel conformation. We dissect the catalytic mechanism with chemical probes and show that ADEP in addition to opening the axial pore directly stimulates ClpP activity through cooperative binding. ClpP activation thus reaches beyond active site accessibility and also involves conformational control of the catalytic residues. Moreover, we demonstrate that substoichiometric amounts of ADEP potently prevent binding of ClpX to ClpP and, at the same time, partially inhibit ClpP through conformational perturbance. Collectively, our results establish the hydrophobic binding pocket as a major conformational regulatory site with implications for both ClpXP proteolysis and ADEP-based anti-bacterial activity. The proper balance of protein synthesis and protein degradation on a cellular level is of pivotal importance in all kingdoms of life and its perturbation is currently intensively investigated for therapeutic application in the context of cancer, inflammation and infectious diseases [1] , [2] , [3] . Recently, two opposite strategies based on the chemical stimulation or inhibition of protein degradation have been shown to either kill bacteria or silence their pathogenesis [4] . β-lactones are covalent inhibitors of the bacterial serine protease ClpP [5] , [6] . Inhibition of ClpP enzymatic activity halts the degradation of proteins involved in virulence regulation, which results in attenuated pathogenesis [7] , [8] . In contrast, ADEPs are a class of natural product-derived cyclic acyldepsipeptides that act as potent antibiotics through the dysregulation and activation of ClpP [9] , [10] . In an unperturbed cell, proteolysis occurs through binding of a AAA+ chaperone such as ClpX to the apical sides of the barrel-shaped, proteolytic component ClpP whereupon a functional ClpXP protease complex with a continuous substrate channel is formed [11] , [12] , [13] , [14] , [15] . In this complex, ClpX engages substrate proteins prone to degradation, unfolds them and threads them into the ClpP proteolytic chamber where they are subsequently degraded [16] , [17] , [18] . Crystal structures of the ClpP barrel in different conformations have been solved, including an active extended and an inactive compressed conformation, however, how the associated structural dynamics are regulated is currently not known [6] , [13] , [19] , [20] . ClpP alone is able to cleave only small peptides, with binding of ClpX being strictly required for the degradation of proteins [21] . ADEPs eliminate this regulation by binding at the junction of the ClpP subunits in a hydrophobic pocket that is also used by ClpX [22] , [23] . Binding of ADEPs causes a conformational change in the N-terminal region of ClpP whereupon the axial pore of the protease is enlarged allowing proteins to access the ClpP active sites within the degradation chamber ( Fig. 1a ) [24] , [25] . Proteomic experiments showed that this uncontrolled proteolysis leads to the depletion of several essential proteins such as the bacterial cytoskeleton protein FtsZ, which in turn causes impaired cell division and ultimately cell death [26] , [27] . Since this unique antibiotic mechanism exploits a cellular machinery and activates it for destruction, ADEPs were recently shown to be active also against bacterial persister cells and established biofilms of pathogenic Staphylococcus aureus [27] . 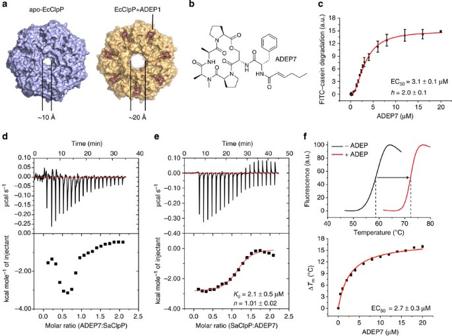Figure 1: ADEP cooperatively binds and stabilizes SaClpP. (a) Binding of ADEP to the hydrophobic pocket on the apical surface of ClpP causes a conformational change that opens the axial substrate entry pore of ClpP (PDB IDs: 1TYF, 3MT6). (b) Structure of ADEP7. (c) ADEP7-induced degradation of FITC–casein by SaClpP (0.5 μM) indicates positive cooperativity (Hill coefficienth=2.0±0.1; EC50=3.1±0.1 μM). (d) ITC titration of ADEP7 (500 μM) into a solution of SaClpP (50 μM) shows positive cooperative binding, which prevents standard data analysis. (e) ITC titration of SaClpP (617 μM) into a solution of ADEP7 (62 μM). Parameters obtained from this experiment are: stoichiometry factorn=1.01±0.02;Kd=2.1±0.5 μM; ΔH=−3369±100 cal mol−1; ΔS=13.8 cal mol−1K−1. The stoichiometry factor refers to the ratio of monomeric SaClpP and ADEP7. A value of 1 is equivalent to 14 ADEP molecules binding per SaClpP14. (f) Thermal shift assays reveal strong stabilization of SaClpP folding by ADEP7 in a concentration-dependent manner (melting temperature of free SaClpP: 58.3 °C; ADEP7 concentration in upper panel: 12 μM; EC50=2.7±0.3 μM). Plotted data incandfare mean±s.d. (N=3). Parameters determined from curve fits inc,eandfare given with fitting errors. Figure 1: ADEP cooperatively binds and stabilizes SaClpP. ( a ) Binding of ADEP to the hydrophobic pocket on the apical surface of ClpP causes a conformational change that opens the axial substrate entry pore of ClpP (PDB IDs: 1TYF, 3MT6). ( b ) Structure of ADEP7. ( c ) ADEP7-induced degradation of FITC–casein by SaClpP (0.5 μM) indicates positive cooperativity (Hill coefficient h =2.0±0.1; EC 50 =3.1±0.1 μM). ( d ) ITC titration of ADEP7 (500 μM) into a solution of SaClpP (50 μM) shows positive cooperative binding, which prevents standard data analysis. ( e ) ITC titration of SaClpP (617 μM) into a solution of ADEP7 (62 μM). Parameters obtained from this experiment are: stoichiometry factor n =1.01±0.02; K d =2.1±0.5 μM; Δ H =−3369±100 cal mol −1 ; Δ S =13.8 cal mol −1 K −1 . The stoichiometry factor refers to the ratio of monomeric SaClpP and ADEP7. A value of 1 is equivalent to 14 ADEP molecules binding per SaClpP 14 . ( f ) Thermal shift assays reveal strong stabilization of SaClpP folding by ADEP7 in a concentration-dependent manner (melting temperature of free SaClpP: 58.3 °C; ADEP7 concentration in upper panel: 12 μM; EC 50 =2.7±0.3 μM). Plotted data in c and f are mean±s.d. ( N =3). Parameters determined from curve fits in c , e and f are given with fitting errors. Full size image Here we show that the conformation of the ClpP barrel is controlled through the hydrophobic pocket on the protease surface. ClpP is arrested in the active, extended conformation on engagement with ADEP or chaperone, which leads to a stimulation of catalytic activity. Our results reveal an additional layer of regulation in the ClpXP system: the link between ClpP barrel conformation and occupation of the allosteric sites. This demonstrates that the allosteric binding pocket of ClpP functions as a conformational switch that not only controls the accessibility of the active sites but also their activity. Characterization of the SaClpP–ADEP interaction We set out to investigate the activation of ClpP from S. aureus (SaClpP) by ADEPs and to analyze the corresponding effects on protease function and conformation. We started by screening a small compilation of ADEP derivatives [28] , which we found to be equally potent in inducing SaClpP proteolysis ( Supplementary Fig. 1a–c ). All biochemical and structural assays were performed with ADEP7 ( Fig. 1b ) unless noted otherwise, which showed a slightly higher affinity than the widely used reference compound ADEP4 towards both C-terminally Strep-tagged and native SaClpP protein ( Supplementary Fig. 1d–f ). Wild-type SaClpP was purified as a tetradecamer with 14 identical ADEP binding sites. A detailed concentration-dependent analysis of ADEP7-induced fluorescein isothiocyanate (FITC)–casein degradation by SaClpP exhibited a sigmoidal behaviour and was thus adequately described by the Hill equation ( Fig. 1c ) [25] , [29] . Data analysis yielded an affinity constant of 3.1 μM and a Hill parameter of 2.0, indicative of positive cooperativity and consistent with previous studies on Escherichia coli ClpP [25] , [29] . Isothermal titration calorimetry (ITC) experiments in which ADEP7 was added to a solution of SaClpP showed nonstandard behaviour [30] ( Fig. 1d ) with the reaction becoming more exothermic during the initial increase of the ADEP7:SaClpP ratio. This can be explained by a lower binding affinity of the initial ADEP molecules and thus confirms positive cooperativity. We next reverted the conditions and titrated SaClpP into a solution of ADEP7 thereby starting with a fully saturated SaClpP ( Fig. 1e ). Here data analysis yielded an ADEP7:SaClpP molar ratio of 1.0 and a K d of 2.1 μM, which likely describes the binding of an ADEP7 molecule to a SaClpP tetradecamer that already has several ADEP molecules bound (see Supplementary Fig. 2 for replicate and control experiments and Supplementary Table 1 for a compilation of parameters obtained from ITC experiments). We further determined the degree of stabilization in a thermal shift assay ( Fig. 1f ). Addition of ADEP7 led to a drastic increase in the protein melting temperature and thus SaClpP folding stability with an half-maximal effective concentration of 2.7 μM. Collectively, these data confirm an affinity of ADEP7 to SaClpP in the 2–3 μM range, slightly higher than the values of 0.82 and 0.37 μM determined for Bacillus subtilis ClpP (BsClpP, Supplementary Fig. 3a ) and E. coli ClpP (EcClpP) [25] , respectively. We therefore compared the binding sites based on available structure and sequence data and identified three residues that were different in SaClpP ( Supplementary Fig. 3b,c ). We generated SaClpP mutant proteins where these three residues were replaced by the corresponding amino acids of BsClpP/EcClpP and found that exchanging histidine 83 for phenylalanine was sufficient for increasing the affinity of SaClpP for ADEP7 to a level comparable to BsClpP ( Supplementary Fig. 3d–f ). Notably, the mutation also caused partial heptamer formation as evidenced by size exclusion chromatography. Importantly, this oligomerization defect was completely abrogated by ADEP7 binding, indicating that ADEPs exhibit conformational control over ClpP. The basis for this conformational control as well as for the observed cooperativity was unknown and we therefore decided to carry out a series of in-depth structural and functional studies. ADEP accelerates ClpP catalysis At first, we investigated how binding of ADEP to SaClpP influences protease catalysis. In a simplified view, the cleavage of a peptide substrate can be described as a two-step process in which first the catalytic serine is acylated by a nucleophilic attack at the scissile amide bond, and second the acyl-ester intermediate is hydrolyzed by a water molecule to regenerate the free enzyme ( Fig. 2a ). To dissect the mechanism of catalysis, we made use of customized β-lactones that were previously described and characterized as SaClpP inhibitors [5] , [31] . These compounds can be viewed as electrophilic, stripped-down substrate mimetics in which the R 1 substituent resembles the S1 amino acid side chain and which otherwise lack an amide backbone or prime site substituents [32] . 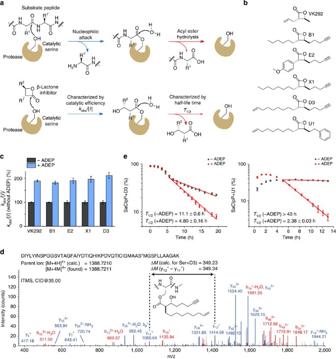Figure 2: ADEP accelerates ClpP catalysis. (a) Simplified schematic representations of the reactions of the SaClpP active site serine with a substrate peptide (upper panel) and with a β-lactone (lower panel). (b) Structures of β-lactones used in this study. (c) Catalytic efficiencies for the reactions of SaClpP (0.5 μM) with five β-lactones in the presence or absence of saturating ADEP7 (12 μM). For each lactone, values were normalized to the respective catalytic efficiency in the absence of ADEP7 for easy comparison. SeeSupplementary Fig. 4for raw data, error bars denote fitting errors. (d) CID fragmentation spectrum of the peptide indicated bearing a covalent modification of β-lactone D3 at the catalytic serine 98 of SaClpP (y ions, blue; b ions, red). For a complete list of identified fragments, referSupplementary Table 2. (e) ADEP7 accelerated the acyl-ester hydrolysis step. SaClpP (10 μM) was incubated for 5 min with saturating concentrations of lactone D3 and U1 (50 μM), then diluted fivefold and treated with ADEP7 (12 μM) or DMSO, followed by incubation at 37 °C. The degree of covalent modification of SaClpP was quantified via intact-protein mass spectrometry after several time points (three independent experiments, mean±s.d.). CID, Collision-Induced Dissociation. Figure 2: ADEP accelerates ClpP catalysis. ( a ) Simplified schematic representations of the reactions of the SaClpP active site serine with a substrate peptide (upper panel) and with a β-lactone (lower panel). ( b ) Structures of β-lactones used in this study. ( c ) Catalytic efficiencies for the reactions of SaClpP (0.5 μM) with five β-lactones in the presence or absence of saturating ADEP7 (12 μM). For each lactone, values were normalized to the respective catalytic efficiency in the absence of ADEP7 for easy comparison. See Supplementary Fig. 4 for raw data, error bars denote fitting errors. ( d ) CID fragmentation spectrum of the peptide indicated bearing a covalent modification of β-lactone D3 at the catalytic serine 98 of SaClpP (y ions, blue; b ions, red). For a complete list of identified fragments, refer Supplementary Table 2 . ( e ) ADEP7 accelerated the acyl-ester hydrolysis step. SaClpP (10 μM) was incubated for 5 min with saturating concentrations of lactone D3 and U1 (50 μM), then diluted fivefold and treated with ADEP7 (12 μM) or DMSO, followed by incubation at 37 °C. The degree of covalent modification of SaClpP was quantified via intact-protein mass spectrometry after several time points (three independent experiments, mean±s.d.). CID, Collision-Induced Dissociation. Full size image The nucleophilic attack of the active site serine at the β-lactone carbonyl leads to ring opening and acylation. We quantified this step by measuring catalytic efficiencies (that is, observed rate constant per inhibitor concentration values, k obs /[ I ]) for five different β-lactones both in the presence and absence of ADEP7 ( Fig. 2b,c , Supplementary Fig. 4 ). The values spanned a range of 3 orders of magnitude and correlated well with the length of the R 1 substituent as established previously [31] . In addition, we confirmed the site of modification by peptide mass spectrometry to be the catalytic serine 98 ( Fig. 2d ). Comparing the catalytic efficiencies in the presence of a saturating amount of ADEP7 to the respective value of free SaClpP yielded a general increase of a factor of 2, irrespective of the size of the β-lactone ( Fig. 2c ). Previous structural studies have revealed that ADEP enlarges the axial pore of ClpP from a diameter of roughly 10 to 20 Å, and pore opening is currently viewed as the sole reason for ADEP activity [24] , [25] . Our data suggest an additional stimulation of catalytic turnover since the increase in catalytic efficiency was found to be independent of the size of the β-lactone inhibitor and was also obtained with the smallest compound VK292, which has a maximum diameter of ~7 Å. To quantitatively assess the second reaction step, the hydrolysis of the acyl-enzyme intermediate, we incubated SaClpP with high concentrations of lactones D3 and U1, diluted the reaction mixture and followed the hydrolysis of the acyl-ester intermediate by intact-protein mass spectrometry both in the presence and absence of ADEP7 ( Fig. 2e ). ADEP again dramatically increased the reaction velocity roughly by twofold by decreasing the half-life time ( T 1/2 ) of the hydrolysis of D3 from 11.1 to 4.8 h. The behaviour of lactone U1 is different in that it reacts more slowly with the enzyme, but once acylation has occurred it exhibits particularly slow hydrolysis ( T 1/2 >40 h). While the reason for this β-lactone-inherent difference is unknown, ADEP7 released this impediment and caused even faster hydrolysis with a T 1/2 of 2.38 h. Since the hydrolysis reaction occurs within the catalytic chamber, the state of the N-terminal residues (that is, the diameter of the axial pore) is not expected to affect the hydrolysis velocity (for coordinated conformational changes, see the Discussion section). Hence these results unequivocally demonstrate allosteric stimulation of ClpP catalytic activity by ADEP, independent of axial pore enlargement. We next examined if this stimulation of activity is accompanied by functional changes of the active site. To this end, we analyzed the turnover of a fluorogenic substrate peptide (Suc-LY-AMC) and observed that saturating ADEP only affected the catalytic rate constant k cat,app , while the affinity constant K M,app remained unchanged ( Supplementary Fig. 5a ). Moreover, we screened a variety of β-lactones with diverse substituents for their potential to acylate SaClpP in the presence and absence of ADEP7; however, ADEP did not apparently change the preference of SaClpP for specific β-lactone probes ( Supplementary Fig. 5b,c ). In addition, we synthesized all four stereoisomers of lactone U1 and looked for changes in binding through intact-protein mass spectrometry. Only the ( S,S )-configured lactone reacted with SaClpP with both cis -configured lactones showing marginal modification of the protease ( Supplementary Fig. 5d,e ). These results indicate that the ADEP-induced increase of catalytic activity is not due to a change in geometry of the ClpP substrate pocket. Consistent with this, previous co-crystal structures of both BsClpP and EcClpP revealed no difference in the orientation of the active site catalytic triad on ADEP1 binding and ascribed the effect of ADEP binding to a change in the nearby N-terminal region [24] , [25] . These observations excluded that ADEP binding induces a re-orientation of active site residues and raises the question of the molecular mechanism of enhanced catalysis. ADEP allosterically controls ClpP barrel conformation An explanation for the unusual ADEP-induced activation in line with all previous experiments would be a stimulation of ClpP through conformational restriction of the complex into a more active form. The ClpP protease is known to be highly dynamic [20] and structural information on SaClpP is available for an active extended [19] , an inactive compact [33] and an inactive compressed [6] conformation [34] . These conformations differ in the height of the barrel (~10 nm for the extended and ~9 nm for the compact and compressed conformations), in the alignment of the catalytic triad residues and in the orientation of the E-helix in the handle region ( Fig. 3a and Supplementary Fig. 6a ). Protein NMR studies with EcClpP [35] have revealed the presence of at least two states in solution, which is supported by molecular dynamics simulations [36] and normal mode analysis [37] suggesting that ClpP samples different conformations. We sought to elucidate the structural basis of ADEP allostery by studying a panel of mutant proteins, which adopt different conformational states. We introduced mutations at all residues of the catalytic triad—S98, H123 and D172 (H123A and H123N proteins showed an increased tendency to aggregation and were therefore excluded from further studies). We also mutated the oligomerization sensor residues R171 and D170 (as well as nearby T169), which engage in inter-ring salt bridging depending on the conformational state and thereby facilitate a functional coupling of tetradecamer formation to the catalytic triad [19] , [38] , [39] . Analytical size exclusion chromatography showed a clustering of these mutants into three distinct groups ( Fig. 3b ). While the R171A and T169A proteins were clearly heptameric as reported previously [19] , [31] , the D172N and D170A proteins migrated only slightly slower than wild-type, tetradecameric SaClpP. 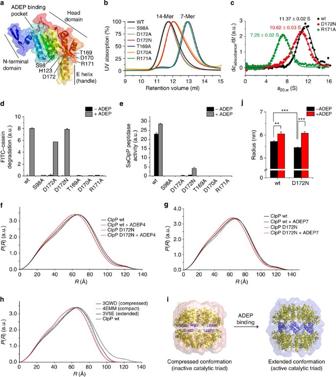Figure 3: Binding of ADEP to ClpP induces a conformational switch to the active, extended ClpP barrel conformation. (a) Cartoon representation of a ClpP monomer showing the position of the ADEP binding site, the catalytic triad (S98, H123, D172) and the oligomerization sensor R171 (PDB ID: 3MT6). (b) Analytical size exclusion chromatograms of wild-type and mutant SaClpP. (c) Analytical ultracentrifugation results for selected mutants. Sedimentation coefficients were obtained as the centres of Gauss functions whose fitting errors are given. (d) FITC–casein degradation activity of wild-type and mutant SaClpP (1 μM) in the presence or absence of ADEP7 (12 μM). Mean±s.d. of initial slopes are given. (e) Peptidase activity of wild-type and mutant SaClpP (0.5 μM) in the presence or absence of ADEP7 (12 μM). Mean±s.d. of initial slopes are given. (f) Inter-atomic pair distance distribution functions (PDDF) of tag-free SaClpP proteins treated with either DMSO or ADEP4 (1:1 mixture, 380 μM, 0.6% DMSO). (g) PDDF of tag-free SaClpP with/without ADEP7 (1:1 mixture, 380 μM, 0.6% DMSO). (h) Comparison of measured (ClpP wt) and predicted (3QWD, 4EMM, 3V5E) inter-atomic pair distance distribution functions. (i)Ab initiolow-resolution models of SAXS scattering curves from SaClpP-D172N superimposed with SaClpP in the compressed conformation (left), as well as from SaClpP-D172N+ADEP4 superimposed with SaClpP in the extended conformation (right). (j) Dynamic light scattering results of wild type and D172N SaClpP treated with either DMSO or ADEP7 (1:1 mixture, 310 μM, 3% DMSO). Please note the axis break. Mean±s.e.m.; **P<0.01, ***P<0.001 (independent two-samplet-tests,N=10, with each of these 10 results established from 10 technical replicates, equal variances not assumed). UV, ultraviolet. We confirmed the integrity of all protein samples by a Coomassie gel as well as by intact-protein mass spectrometry to exclude abnormal autocatalytic processing ( Supplementary Table 3 ). We also confirmed the assigned oligomerization states by size exclusion chromatography–multiangle light scattering (SEC–MALS) analysis ( Supplementary Fig. 6b ). In addition, we validated these data by analytical ultracentrifugation, which also indicated a different sedimentation of the D172N mutant compared with wild-type SaClpP ( Fig. 3c ). With the molecular masses of the subunits as well as the oligomerization unchanged, the smaller appearance in the size exclusion experiment of D172N proteins could result from a more compact/compressed tetradecameric conformation. Figure 3: Binding of ADEP to ClpP induces a conformational switch to the active, extended ClpP barrel conformation. ( a ) Cartoon representation of a ClpP monomer showing the position of the ADEP binding site, the catalytic triad (S98, H123, D172) and the oligomerization sensor R171 (PDB ID: 3MT6). ( b ) Analytical size exclusion chromatograms of wild-type and mutant SaClpP. ( c ) Analytical ultracentrifugation results for selected mutants. Sedimentation coefficients were obtained as the centres of Gauss functions whose fitting errors are given. ( d ) FITC–casein degradation activity of wild-type and mutant SaClpP (1 μM) in the presence or absence of ADEP7 (12 μM). Mean±s.d. of initial slopes are given. ( e ) Peptidase activity of wild-type and mutant SaClpP (0.5 μM) in the presence or absence of ADEP7 (12 μM). Mean±s.d. of initial slopes are given. ( f ) Inter-atomic pair distance distribution functions (PDDF) of tag-free SaClpP proteins treated with either DMSO or ADEP4 (1:1 mixture, 380 μM, 0.6% DMSO). ( g ) PDDF of tag-free SaClpP with/without ADEP7 (1:1 mixture, 380 μM, 0.6% DMSO). ( h ) Comparison of measured (ClpP wt) and predicted (3QWD, 4EMM, 3V5E) inter-atomic pair distance distribution functions. ( i ) Ab initio low-resolution models of SAXS scattering curves from SaClpP-D172N superimposed with SaClpP in the compressed conformation (left), as well as from SaClpP-D172N+ADEP4 superimposed with SaClpP in the extended conformation (right). ( j ) Dynamic light scattering results of wild type and D172N SaClpP treated with either DMSO or ADEP7 (1:1 mixture, 310 μM, 3% DMSO). Please note the axis break. Mean±s.e.m. ; ** P <0.01, *** P <0.001 (independent two-sample t -tests, N =10, with each of these 10 results established from 10 technical replicates, equal variances not assumed). UV, ultraviolet. Full size image To correlate ClpP conformations with both peptidase and proteolytic activity, we functionally characterized the mutant enzymes in the presence of ADEP ( Fig. 3d,e ). Both mutants of the active site aspartate (D172A and D172N) containing a weakened charge-relay system of the catalytic triad were catalytically inactive alone. Unexpectedly, they gained proteolytic activity in the presence of ADEP, with undistinguishable activity of D172N and wild type in a FITC–casein degradation assay. Moreover, ADEP stimulated hydrolysis of the fluorogenic peptide Suc-LY-AMC in the D172N but not in the D172A mutant. We speculated that subtle changes near the oligomerization sensor residues of ClpP such as D172N might trigger the adoption of a compacted conformation as the lowest energy state. To investigate the mutation- and ADEP-induced changes in more detail on a structural level, we applied small angle X-ray scattering (SAXS; Fig. 3f,g ). A comparison of the inter-atomic pair distance distribution functions (PDDF, P ( R )) of wild-type and D172N SaClpP clearly showed a more compacted conformation of the D172N protein. The data also demonstrate that the oligomeric assemblies in wild-type and D172N SaClpP have the same mass (identical integral of the P ( R ) in Fig. 3f , see Table 1 ), confirming different conformations rather than oligomerization states. Addition of either ADEP4 or ADEP7 led to an increase in the size of both the wild-type and the D172N protein as revealed by a shift in the P ( R ) function, and the conformations became virtually indistinguishable in the ADEP-bound state. The ADEP-induced shift of the P ( R ) function as well as of the radius of gyration, R g , in the D172N sample is fully in agreement with the shift predicted by analyzing the structures of the compressed and the extended conformation ( Fig. 3h ; Δ R g (compressed->extended),calculated =1.8 Å;Δ R g (SaClpP-D172N->+ADEP4), observed =1.7 Å). Moreover, low-resolution models inferred from the data support the conclusion of an ADEP-mediated shift from a compressed to an extended conformation in the D172N protein ( Fig. 3i ). Notably, also the wild-type protein either bound to ADEP4 or ADEP7 showed a small increase in size. The inter-ring bridge mutants T169A and R171A were clearly heptameric in SAXS analysis and failed to assemble to functional tetradecameric complexes on addition of ADEP, which is in line with their lack of catalytic activity ( Supplementary Fig. 6c–f ). SAXS data were recorded three times with independently purified protein samples including tag-free and C-terminally Strep-tagged protein, and the described changes were consistently visible. Table 1 SAXS data and analysis of SaClpP proteins. Full size table It has been speculated that the compressed conformation precludes ADEP binding due to a closed binding pocket [33] . Consistently, we found a rough threefold lower affinity of SaClpP-D172N for ADEP7 by ITC while the affinity towards SaClpP-S98A was less affected ( Supplementary Fig. 2e,f ). In addition, we validated the SAXS results with dynamic light scattering (DLS), which significantly showed a small ADEP-induced increase in the wild-type protein radius and a larger ADEP-induced increase in the D172N sample, with both ADEP-bound proteins being equal in size ( Fig. 3j ). Since it is difficult to correlate static crystal structures to the data inferred from solution-based methods, the possibility remains that the compressed structure we are observing in solution may not entirely represent that described by X-ray crystallography. However, when taken together, these data clearly demonstrate how binding of ADEP exhibits conformational control on the ClpP barrel. Occupation of the regulatory allosteric site reverts the catalytically incompetent, compressed conformation of the D172N mutant and locks the wild-type protein in an extended conformation, explaining the ADEP-induced increase in catalytic activity. Substoichiometric occupation leads to partial inhibition When we analyzed the concentration-dependent response of SaClpP peptidase activity to ADEP7, we unexpectedly found biphasic behaviour. While saturating amounts of ADEP stimulated SaClpP peptidase activity as described above, small ADEP concentrations corresponding to three to four ADEP molecules per SaClpP 14 showed partial inhibition ( Fig. 4a ). This partial inhibition was also observed with ADEP4, as well as with tag-free SaClpP protein ( Supplementary Fig. 7a–c ). Moreover, a similar phenomenon was observed with the D172N mutant whose low residual peptidase activity was further diminished by adding a small amount of ADEP ( Fig. 4b ). Consistent with the wild-type SaClpP data, no such effect was observed during proteolysis ( Fig. 4c ). We analyzed the respective SaClpP:ADEP ratios via analytical ultracentrifugation and found that a substoichiometric amount of ADEP slightly decreased the sedimentation coefficient of wild-type ClpP, whereas this effect was reverted at higher ADEP concentrations ( Fig. 4d ). Similarly, the sedimentation coefficient of D172N first decreased with small amounts of ADEP and increased to a higher value than the free protein on further addition of ADEP ( Fig. 4e ). We hypothesize that binding of the initial ADEP molecules to a tetradecameric ClpP induces structural perturbations owing to a conformationally heterogeneous assembly, which would also account for the observed positive cooperativity. 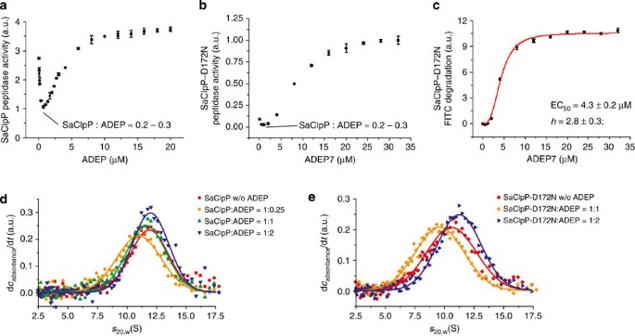Figure 4: Substoichiometric amounts of ADEP cause partial inhibition of ClpP. (a) Concentration-dependent partial inhibition or stimulation of wild-type SaClpP peptidase activity by ADEP7. The ratio of ADEP bound to ClpP was estimated from the concentrations at the minimum and aKdof 2.1 μM. A ratio of 0.2–0.3 corresponds to 2.8–4.2 ADEP molecules per SaClpP14. (b) Concentration-dependent inhibition or stimulation of SaClpP-D172N peptidase activity by ADEP7. In line with the compressed conformation of SaClpP-D172N, the initial peptidase activity is lower than that of the wild-type protein. The ratio of ADEP bound to ClpP was estimated from aKdof 6.1 μM. (c) FITC–casein degradation by SaClpP-D172N indicates positive cooperativity (h=2.8±0.3; EC50=4.3±0.2 μM). (d) Analytical ultracentrifugation results of SaClpP (7.5 μM) treated with DMSO (0.6% (v/v)) or ADEP7 (2, 7.5 and 15 μM). (e) Analytical ultracentrifugation results of SaClpP-D172N (7.5 μM) treated with DMSO (0.6% (v/v)) or ADEP7 (7.5 and 15 μM). Plotted data ina–care mean±s.d. (N=3). Parameters determined from curve fits incare given with fitting errors. Figure 4: Substoichiometric amounts of ADEP cause partial inhibition of ClpP. ( a ) Concentration-dependent partial inhibition or stimulation of wild-type SaClpP peptidase activity by ADEP7. The ratio of ADEP bound to ClpP was estimated from the concentrations at the minimum and a K d of 2.1 μM. A ratio of 0.2–0.3 corresponds to 2.8–4.2 ADEP molecules per SaClpP 14 . ( b ) Concentration-dependent inhibition or stimulation of SaClpP-D172N peptidase activity by ADEP7. In line with the compressed conformation of SaClpP-D172N, the initial peptidase activity is lower than that of the wild-type protein. The ratio of ADEP bound to ClpP was estimated from a K d of 6.1 μM. ( c ) FITC–casein degradation by SaClpP-D172N indicates positive cooperativity ( h =2.8±0.3; EC 50 =4.3±0.2 μM). ( d ) Analytical ultracentrifugation results of SaClpP (7.5 μM) treated with DMSO (0.6% (v/v)) or ADEP7 (2, 7.5 and 15 μM). ( e ) Analytical ultracentrifugation results of SaClpP-D172N (7.5 μM) treated with DMSO (0.6% (v/v)) or ADEP7 (7.5 and 15 μM). Plotted data in a – c are mean±s.d. ( N =3). Parameters determined from curve fits in c are given with fitting errors. Full size image Despite a sequence homology of ~60% ( Supplementary Fig. 3b ), ClpP proteins from different species are remarkably different in their oligomerization behaviour. We studied BsClpP, which under our purification conditions using affinity and size exclusion chromatography in glycerol containing buffer yielded a tetradecameric and a monomeric fraction ( Supplementary Fig. 7d–i ) [10] . In analogy to SaClpP, the intrinsically active tetradecameric BsClpP showed partial inhibition of peptidase activity at low ADEP concentrations while the monomeric BsClpP was inactive in the absence of ADEP and was activated with an even lower ADEP concentration than the tetradecameric BsClpP ( Supplementary Fig. 7e–g ). Similar results were obtained with Listeria monocytogenes ClpP2 (LmClpP2) tetradecamer and heptamer ( Supplementary Fig. 7h,i ) [40] . These data provide evidence that the hydrophobic ADEP binding pocket acts as a major conformational regulatory site across organisms, which allows for differential regulation of protease activity depending on the degree of occupation per tetradecamer. SaClpX and ADEP share a ClpP activation mechanism The ADEP-bound conformation of ClpP has been suggested to serve as a model for the Clp–ATPase-bound state of ClpP since ADEP and the IGF loop of ClpX are assumed to share the same binding site. We therefore reasoned that ClpX might be able to exert conformational control on ClpP in a similar way. We thus tested all protein mutants in a SaClpXP assay in which we monitored the fluorescence of a green fluorescent protein (GFP) variant to which a C-terminal degradation tag (SsrA tag) was appended ( Fig. 5a,b ) [17] . To differentiate between GFP unfolding and degradation, the assay mixture was analyzed by Coomassie gel after 3 h. The D172N mutant showed GFP degradation activity similar to the wild-type enzyme, which is in full agreement with the results of ADEP-induced casein degradation, indicating that SaClpX is also able to revert the compressed conformation of the D172N protein. The intermediate assay signal of the S98A mutant protein was assigned as unfolding activity without proteolysis [41] , whereas the heptameric oligomerization of the T169A and R171A mutants consistent with the SAXS data precluded activation by SaClpX and thus GFP unfolding. In a competition assay, ADEP7 and ADEP4 inhibited GFP unfolding by SaClpXP and thus binding of SaClpX to ClpP with IC 50 values of 225 and 221 nM ( Fig. 5c ). This value is in the range of the assay concentration of tetradecameric SaClpP (200 nM), consistent with a shared binding site of ADEP and ClpX [10] . The IC 50 , furthermore, suggests that the binding of a single ADEP molecule to only one SaClpP apical surface is sufficient to reduce SaClpXP proteolysis by half ( Fig. 5e ). 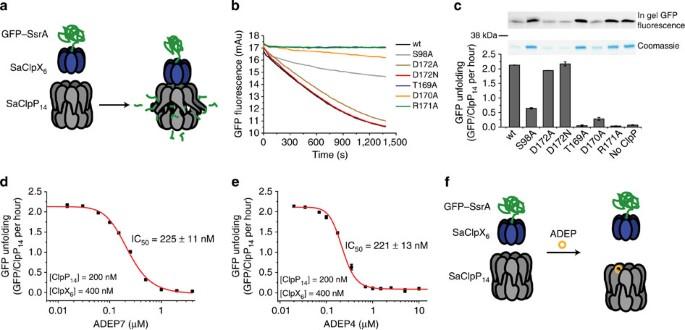Figure 5: ClpX activates ClpP in a similar manner and is competed by ADEP. (a) Schematic of the SaClpX-mediated unfolding of SsrA-tagged GFP and its subsequent degradation by SaClpP. (Note, the precise path of product peptide release is unclear and under debate.) (b) SaClpXP–GFP assay. The initial slopes of the decrease in GFP fluorescence of the fluorescence-time courses were quantified and are displayed in the bar graph. A Coomassie-stained gel of these samples showing GFP after 3 h at 30 °C indicates that wild-type, D172A, D172N, and D170A SaClpP are capable of protein degradation, while S98A, T169A and R171A SaClpP are not. This is consistent with in-gel GFP fluorescence measurements. SeeSupplementary Fig. 7n,ofor uncropped gel images. (c,d) ADEP7 and ADEP4 disrupt SaClpXP-mediated GFP unfolding with an IC50value comparable to the concentration of SaClpP14. (e) Schematic showing how the binding of ADEP to SaClpP14prevents the binding of ClpX6and thus GFP unfolding. Mean±s.d. are given in all panels (N=3). IC50values are given with fitting errors. Figure 5: ClpX activates ClpP in a similar manner and is competed by ADEP. ( a ) Schematic of the SaClpX-mediated unfolding of SsrA-tagged GFP and its subsequent degradation by SaClpP. (Note, the precise path of product peptide release is unclear and under debate.) ( b ) SaClpXP–GFP assay. The initial slopes of the decrease in GFP fluorescence of the fluorescence-time courses were quantified and are displayed in the bar graph. A Coomassie-stained gel of these samples showing GFP after 3 h at 30 °C indicates that wild-type, D172A, D172N, and D170A SaClpP are capable of protein degradation, while S98A, T169A and R171A SaClpP are not. This is consistent with in-gel GFP fluorescence measurements. See Supplementary Fig. 7n,o for uncropped gel images. ( c , d ) ADEP7 and ADEP4 disrupt SaClpXP-mediated GFP unfolding with an IC 50 value comparable to the concentration of SaClpP 14 . ( e ) Schematic showing how the binding of ADEP to SaClpP 14 prevents the binding of ClpX 6 and thus GFP unfolding. Mean±s.d. are given in all panels ( N =3). IC 50 values are given with fitting errors. Full size image Multicomponent protease complexes require the precise coordination of several processes including substrate engagement, unfolding, degradation and product release. To this end, the different parts of the complexes need to be functionally coupled in an accurate and versatile manner. Moreover, information must be coded in structural form and transmitted through allosteric binding events. Since uncontrolled proteolysis poses a threat to cellular viability, reliable and multi-layered regulation is essential for these machineries. The ClpXP protease is a prime example of such a complex since the dynamics of its components have been studied and a framework of reference structures exist [42] , [43] , though a structure of the entire complex is lacking [34] , [44] , [45] , [46] . Biochemical experiments have shown that ClpX interacts with ClpP primarily through docking of its IGF loop into a hydrophobic pocket on the surface of ClpP that is also used by ADEPs to dysregulate ClpP [22] , [23] , [24] . The N-termini of ClpP have been shown to gate the entry into the degradation chamber by adopting different conformations, where the ‘down’ conformation as a hydrophobic plug closes and the ‘up’ conformation opens the entry portal [47] , [48] . Although ADEPs have already been shown to regulate these gated pores, further activating influences of the antibiotic had not been considered. Here we show that ADEPs additionally stimulate ClpP catalysis through cooperative binding. In previously published studies on ADEP-ClpP co-crystal structures this allosteric activation had been missed, since it is not based on changes of active site geometry but on conformational dynamics. We find that ADEPs are able to revert the catalytically incompetent compressed conformation of the D172N ClpP mutant through switching its conformation to the extended state, which exhibits an aligned catalytic triad (contrary to the compressed conformation, where the triad is not aligned). Similarly, ClpX activates ClpP-D172N for proteolysis, implicating that a chaperone is also able to induce the conformational switch of the ClpP-D172N barrel conformation necessary for catalysis. Importantly, we observe that also wild-type ClpP adopts an extended state by addition of ADEP. Our biochemical and structural data thus converge at the view that occupation of the hydrophobic pocket arrests the dynamic ClpP barrel in its catalytically competent conformation, which contributes to sustained peptidase as well as proteolytic activity. Conformational arrest [49] , [50] is a strong regulation principle in ClpP as it even compensates for the lack of a catalytic D172 residue and facilitates proteolytic processing with a Ser–His catalytic dyad. This interpretation is corroborated by a previous study on functional coupling in the ClpXP complex, where occupation of the ClpP active site by a covalent inhibitor increased the affinity of the peptidase for the ATPase [22] . Our results now establish the bidirectionality of this cross-talk and implicate ClpP conformations and catalytic activity in this regulation. Studies on the human ClpP [51] , [52] showed that hClpP is heptameric in solution and that its catalytically competent tetradecameric state can be triggered by addition of ClpX from E. coli [53] . These data suggested a conformational coupling of the hydrophobic pocket with the handle domain. Our data structurally expand this finding, showing that this conformational control is also present within tetradecameric ClpP. Further indications came from hydrogen-exchange mass spectrometry experiments where ADEPs were used as ClpX mimetics and ADEP binding induced rigidification of ClpP in the equatorial handle region [48] . Moreover, mutations in the N-terminal region were used to propose that substrate access might coordinate with protease active site reactivity [54] . Most recently, ADEP was shown to contribute to ClpP activation in the heterooligomeric ClpP1P2 system from Mycobacterium tuberculosis , but only in the presence of an additional activating peptide [55] . ClpX interacts with ClpP via two distinct loop structures. ADEP is an IGF-loop model that demonstrates the sophisticated mechanism by which the ATPase exerts conformational control on the peptidase. The hydrophobic pocket at the surface of ClpP serves as the major regulatory ‘button’ that the IGF loop presses to stabilize the extended, catalytically active conformation of ClpP and simultaneously to put the N-terminal loops of ClpP in the upward position [56] , thereby opening the gated pore. Shielding the open ClpP pore with its own pore-2 loops, ClpX establishes a secluded channel for substrate passage into the catalytic cavity. Coupling the two conformational movements to the same allosteric site and regulatory event ensures that catalytic triads are only active, when the pore is securely covered. The ClpXP complex is not homogeneous during operation. In addition to the symmetry mismatch of hexameric ClpX and the axially heptameric ClpP, ClpX was shown to exhibit conformational heterogeneity based on the nucleotide state of the ATPase domain where coordinated hydrolysis by two to four subunits is coupled to substrate translocation [57] , [58] . While we provide evidence that full occupation of the allosteric site on ClpP leads to activation, we also show that a smaller degree of occupation causes partial inhibition through conformational perturbation. It is currently unclear how the symmetry-mismatched interaction of ClpX and ClpP is mediated and how many hydrophobic pockets on one apical side of a ClpP heptamer are occupied by one ClpX hexamer. We find it intriguing that in a SaClpXP assay with concentrations corresponding to two ClpX hexamers bound to the two apical sides of ClpP (that is, a ClpX 6 :ClpP 14 :ClpX 6 complex as observed with electron microscopy) [53] , [59] , [60] , the addition of one ADEP molecule per ClpP tetradecamer was sufficient to reduce the substrate unfolding activity by half ( Fig. 5c,d ). This suggests that occupation of already one of the seven hydrophobic pockets on a ClpP ring is incompatible with ClpX binding, either through cooperativity-induced conformational heterogeneity or through direct collision with ClpX. Moreover, we are fascinated by the unexpected finding that an allosteric activator molecule is also capable of reducing the activity of the catalytic complex when binding at substoichiometric conditions. This allows for a putative model in which ClpP activity is differentially regulated dependent on the respective ClpX binding state. While the relevance of this phenomenon in ClpXP proteolysis is unclear, we find it important to note that low concentrations of ADEP in a medicinal setting may lead to partial ClpP inhibition and thus bacteria with reduced pathogenicity [7] . Collectively, our results shed light on the way ClpP reciprocates activation by ClpX and ADEP. We provide mechanistic insights into how ADEPs and chaperones exhibit conformational control on ClpP and how this interaction goes beyond active site accessibility, but also influences protease catalysis. We provide evidence that the hydrophobic pocket acts as a major regulatory site of ClpP and that the binding of ADEP or ClpX to this site allows for differential regulation of protease activity and conformation depending on the degree of occupation per tetradecamer. Further experiments should investigate if this allosteric layer of regulation is present also in other multicomponent proteases such as the proteasome. Cloning and protein purification C-terminally Strep-tagged ClpP from S. aureus NCTC 8325 (SaClpP) [19] and ClpP from L. monocytogenes (LmClpP2) [40] were purified through affinity and size exclusion chromatography from expression in E. coli BL21(DE3). Tag-free wild-type SaClpP was purified through anion exchange, hydrophobic interaction and size exclusion chromatography [39] . Expression constructs of mutant proteins were created using the QuikChange methodology using primers listed in the Supplementary Table 4 (refs 19 , 39 ). Expression was carried out in BL21(DE3) or SG1146a cells and purification proceeded as described for the wild-type proteins. Strain SG1146a was a gift from S. Gottesman (NIH, Bethesda, USA). Monomeric concentrations of ClpP are given unless otherwise noted. BsClpP was expressed and purified as follows. E. coli SG1146a was transformed with pClpP11 (ref. 61 ). Cultures (1 l) were grown at 37 °C until an OD 600 of 0.4–0.6 was reached. Then expression of the C-terminal His-tagged fusion protein was induced with 1 mM isopropyl-β-D-thiogalactoside and cultures were grown at 28 °C over night. Cells were lysed in buffer A (50 mM sodium phosphate, 300 mM NaCl, 20% (v/v) glycerol, 20 mM imidazole; pH 8.0) using a Precellys homogenisor (PeqLab). Supernatants were mixed with Ni-NTA matrix (Qiagen) at 4 °C over night and subjected to plastic columns (Thermo Scientific). ClpP was eluted with buffer B (50 mM sodium phosphate, 300 mM NaCl, 20% (v/v) glycerol, 250 mM imidazole; pH 8.0). The eluted proteins were concentrated with Amicon Ultra Centrifugal Filters with 10 kDa cutoff (Merck-Millipore) and subjected to gel filtration on an ÄKTA purifier system with a Superdex 200 16/60 column (GE Healthcare). Tetradecamers and monomers of ClpP were eluted with buffer C (50 mM sodium phosphate, 300 mM NaCl, 20% (v/v) glycerol; pH 8.0). Our reported purifications of BsClpP in the absence of glycerol and in the presence of dithiothreitol (DTT) [61] yielded predominately monomeric ClpP [62] . In the presence of glycerol, both tetradecameric and monomer species were obtained ( Supplementary Fig. 7d ). Monomeric BsClpP could be converted to tetradecameric BsClpP through addition of ADEP ( Supplementary Fig. 7h,i ). Enhanced GFP tagged for ClpXP degradation, enhanced GFP–ssrA (eGFP–ssrA), originates from eGFP (protein ID C5MKY7) and was cloned as a fusion protein with an ssrA tag (AANDENYALAA) at the C terminus. An expression clone was assembled using the Gateway cloning strategy (Invitrogen) with pDonr201 as donation vector and pDest007 (ref. 63 ) as expression vector. The expression construct was transformed into E. coli KY2266 cells. Expression was carried out in 4 l LB media after induction with anhydrotetracycline (0.2 mg/l) at an OD 600 of 0.5 for 4 h at 37 °C. The pellet was washed with PBS and resuspended in ice-cold lysis/wash buffer (100 mM Tris, 150 mM NaCl, 1 mM EDTA, pH 8.0). The cells were lysed using a Constant Cell Disruption system. The lysate was cleared via centrifugation (38,000 g, 45 min, 4 °C). Protein purification was achieved on an Äkta Purifier 10 system (GE Healthcare). Affinity chromatography was carried out with a StrepTrap HP 5 ml column. eGFP–ssrA containing elution fractions were pooled, concentrated and purified with a HiLoad 16/60 Superdex 200 pg gel filtration column in GF buffer (100 mM NaCl, 20 mM Tris, 10% (v/v) glycerol, pH 7.0). Tag-free ClpX from S. aureus NCTC 8325 (SaClpX) was used in all experiments and obtained as follows. The gene encoding ClpX (geneID 3919696) was amplified using primers listed in Supplementary Table 4 . An expression construct was assembled using the Gateway cloning strategy with pDonr207 as donation vector and pET300 as expression vector. The expression construct encoding N-terminally His 6 -tagged, full-length SaClpX with an N-terminal TEV site was transformed into chemically competent BL21(DE3) cells. Expression was carried out in 1 l LB media after induction with isopropyl-β-D-thiogalactoside (0.5 mM) at an OD 600 of 0.6 for 15 h at 25 °C. The cell pellet was washed with PBS and resuspended in ice-cold lysis buffer (50 mM Hepes pH 7.5, 300 mM KCl, 15% (v/v) glycerol, 1 mM DTT). The cells were lysed with a Constant Cell Disruption system and subsequent sonification (3 × 30 s, 80%, Bandelin sonoplus). MgCl 2 (5 mM) was added and the suspension was cleared through centrifugation (36,000 g , 30 min, 4 °C). Affinity purification was carried out on an ÄKTA Purifier 10 chromatography system with a Ni-NTA Superflow cartridge (5 ml). The column was equilibrated in lysis buffer (+5 mM MgCl 2 ), the lysate was loaded and it was washed with 10 column volumes lysis buffer (+ 5 mM MgCl 2 ,+40 mM imidazole). Elution was carried out with a steep gradient in elution buffer (lysis buffer+5 mM MgCl 2 +500 mM imidazole). EDTA (2 mM) and TEV protease (500 μl of 1.7 mg ml −1 stock) were added to the pooled elution fractions and it was incubated at 4 °C over night. Cleavage was monitored by intact-protein mass spectrometry and SDS–PAGE. If necessary, a second addition of TEV protease was carried out followed by incubation at 4 °C over night. The sample was concentrated with a 10 kDa Amicon ultra centrifugal filter to reduce the imidazole content, diluted in breaking buffer (10 ml final volume, final imidazole: 40 mM). MgCl 2 (2 mM) was added and the solution was passed through a pre-equilibrated Ni-NTA column. The flow-through was collected, three times buffer-exchanged with a 10 kDa Amicon ultracentrifugation device in lysis buffer (+ 2 mM MgCl 2 ) and frozen in aliquots. A gel filtration step was omitted since analytical runs showed no signs of aggregated protein. Peptidase activity assay ADEP (1 μl of 100 × stock in dimethylsulphoxide (DMSO)) was placed into black flat-bottom 96-well plates. Solutions of SaClpP (90 μl, final concentration: 0.5–1 μM) in assay buffer E (100 mM Hepes pH 7.0, 100 mM NaCl) were added and incubated at 32 °C for 15 min. Then Suc-LY-AMC solution (10 × , final concentration: 200 μM; also preheated to 32 °C) in assay buffer B was added to the wells (10 μl each, assay volume: 100 μl). The reaction was monitored by following the increase of fluorescence (excitation: 380 nm, emission: 440 nm), which was recorded with one measurement per minute using an infinite M200Pro plate reader (Tecan) at 32 °C. Slopes were calculated with Microsoft Excel from the fluorescence over time plots via linear regression, whereby a 5-min lag period at the beginning of the measurement was excluded. All data were recorded in triplicate and in at least two independent experiments. S.d. was calculated from triplicate measurements. Normalization was achieved through measurement of the fluorescence of a set of completely cleaved Suc-LY-AMC samples with different concentrations (0.2–6 μM). LmClpP2 assay buffer (100 mM Hepes pH 7.0, 100 mM KCl) was used for LmClpP2 activity measurements with addition of glycerol (15% v/v) where indicated. BsClpP assay buffer (50 mM Tris-HCl, 25 mM MgCl 2 , 100 mM KCl, 2 mM DTT; pH 8.0) was used for BsClpP activity measurements (1 μM BsClpP; 100 μl reaction volume; 0.5 μl DMSO/ADEP 200 × ; excitation/emission: 380/460 nm). Catalytic efficiency measurements Serial β-lactone inhibitor dilutions (1 μl of 100 × stock in DMSO) were added to wells and Suc-LY-AMC (50 μl, 2 × , final concentration: 200 μl) in assay buffer A was added. ADEP (12 μM from 10 mM stock) or the respective amount of DMSO was added to a SaClpP solution (2 × , final concentration: 1 μM) in assay buffer A and everything was brought to 32 °C. Subsequently, 50 μl of the protein solution was added to the wells and fluorescence was recorded as described above with a 20-s interval. Kinetic constants were obtained assuming pseudo-first-order kinetics by fitting the curves to wherein F ( t ) denotes the fluorescence-time course, F 0 denotes the initial fluorescence, A denotes the slope of the uninhibited control samples and k obs denotes the rate constant. Catalytic efficiencies were determined as slopes from k obs /[ I ] plots [31] . FITC–casein assay ADEP (1 μl of 100 × stock in DMSO) was added to wells of black flat-bottomed 96-well plates. Protein dilution (80 μl, 1.2 × , final concentration: 1 μM) was added and incubated at 37 °C for 15 min. Casein mix (20 μl, 5 × , final concentration of mixed casein: 0.24 mg ml −1 , final concentration of FITC–casein: 0.048 mg ml −1 ) was added and the reaction was followed in an infinite M200Pro plate reader with excitation at 494 nm and detection at 521 nm at 37 °C. Initial slopes (usually 0–300 s) were used for data analysis. All data were referenced against the slope of casein solution without addition of protease. Fitting was performed with OriginPro (Microcal) using the Michaelis–Menten equation, wherein instead of a K m the half-maximal effective concentration EC 50 was used. Isothermal titration calorimetry All ITC experiments were performed on a MicroCal iTC200 system (GE Healthcare) in 20 mM Hepes pH 7.0, 100 mM NaCl with a maximum of 2% (v/v) DMSO at 25 °C and with constant stirring at 1,000 r.p.m. Prior to experiments, the protein was gel filtrated into 20 mM Hepes pH 7.0, 100 mM NaCl, concentrated if necessary using 10 kDa Nanosep centrifugational devices (Pall) and the ligand was dissolved in the exact same buffer from a 50 mM stock in DMSO. DMSO concentrations of syringe and cell samples were matched if necessary by addition of pure DMSO. The experiment was started after equilibration for 300 s with a first injection of 0.4 μl that was discarded during the analysis. A typical experiment consisted of 20 subsequent injections with a 2 μl injection volume into a cell filled with 200 μl sample. Each injection was made over a period of 4 s with a 2–3-min interval between subsequent injections. Power was recorded at ‘high’ gain setting, with a reference power of 10 μcal s −1 and a 5-s filter period. Data analysis including baseline correction and evaluation was carried out with OriginPro 8.5ITC. Due to cooperativity and thus the nonstandard form of some ITC curves, no fits based on simplified models were obtained for ligand into protein experiments. In the case of protein into ligand experiments, fits were carried out taking into account all injections until the maximum heat occurred and the two subsequent injections. We assume this to reflect the binding of ADEP to a ClpP protein with already some ADEP molecules bound. The binding characteristics of the initial ADEP molecules binding to free ClpP are likely to be different. Thermal shift assay ADEP (0.5 μl of 100 × stocks in DMSO) was placed into wells of white 96-well PCR plates. Sypro Orange (1 × ) was added to a SaClpP (1 μM) solution in buffer D and 50 μl were added to each well. The plate was sealed and fluorescence was recorded in a CFX96 Real-Time System (Bio-Rad) while heating from 20 to 80 °C in 0.3 °C steps. Data analysis was performed with CFX Manager software and OriginPro. Melting temperatures were referenced against the melting temperature of DMSO-treated SaClpP. Intact-protein mass spectrometry Samples were diluted down to 1–2 μM protein concentration in buffer D. Aliquots (4–2 μl) were desalted with a Massprep on-line desalting cartridge (Waters) according to the manufacturer’s procedure on a Dionex UltiMate 3000 HPLC system and subsequently measured on a Thermo LTQ FT Ultra mass spectrometer with electron spray ionization. Promass Deconvolution software (Thermo Scientific) was used for data analysis and deconvolution (input range: 500–2,000 m/z ; output range: 20,000–30,000 Da; peak width=3; merge width=0.3; smooth width=7; number of smooths=2). Thermo Scientific Xtract software was used for verification. For the time-course experiments, SaClpP (10 μM) was incubated for 5 min at room temperature with saturating concentrations of lactone D3 and U1 (50 μM). It was then diluted fivefold and treated with ADEP7 (12 μM) or DMSO, followed by incubation at 37 °C. The degree of covalent modification of SaClpP was quantified via intact-protein mass spectrometry after several time points (three independent experiments). Mass intensities were normalized against the sum of intensities of the free protein and the modified protein. T 1/2 was calculated from linear fits of the logarithmic plots. SEC–MALS Analytical size exclusion chromatography was carried out on an ÄKTA Purifier 10 chromatography system with a calibrated Superdex 200 10/300 GL column in buffer D (20 mM Hepes pH 7.0, 100 mM NaCl) at 4 °C with a flow of 0.5 ml min −1 . Samples (300 μl of a 1 mg ml −1 SaClpP solution or 1 ml of a 250 μg ml −1 solution) were loaded into a 500 μl or 1 ml sample loop and elution was monitored by ultraviolet absorption at 280 nm. Ultraviolet traces were referenced against the salt peak in the conductivity trace and normalized to the highest signal for easy comparison. SEC–MALS analysis was carried out on an Agilent 1200 Series chromatography system equipped with a Superdex 200 10/300 GL column and coupled to a DAWN Heleos II MALS detector as well as a Optilab rEX refractive index detector (Wyatt Technology). Samples (100 μl of 2 mg ml −1 protein solutions) were loaded from an autosampler and analyzed in buffer D (20 mM Hepes pH 7.0, 100 mM NaCl; used for SaClpP proteins and LmClpP2) with a flow of 0.5 ml min −1 or in buffer F (50 mM Tris pH 8.0, 200 mM NaCl, 20% glycerol; used for LmClpP2+glycerol and BsClpP proteins) with a flow of 0.4 ml min −1 . Masses and errors were derived from analysis in Astra 6.1 (Wyatt Technology) and calibration with BSA. Analytical ultracentrifugation Sedimentation velocity experiments were performed in a ProteomeLab XL-A (Beckman Coulter, USA) instrument equipped with a ultraviolet/visible-detection unit. Protein was detected at 280 nm. Runs were performed at 34,000 r.p.m. (93,220 g ) at 20 °C. Proteins were spun in a Ti50 rotor equipped with seven sample cells and one reference counterbalance cell. Samples of mutant and wild-type SaClpP were analyzed in buffer D with different concentrations (7.5–80 μM). Samples of mutant and wild-type SaClpP with ADEP were analyzed in buffer D+0.6% (v/v) DMSO with a protein concentration of 7.5 μM. Scanning intervals were set to 0.003 cm. All data were verified by at least two independent experiments. Data analysis was performed using the ‘Time Course’ function of the SedView programme. In addition, all the sedimentation experiments were evaluated with the UltraScan II software. Small angle X-ray scattering SAXS data for solutions of SaClpP wild-type and mutant samples free and bound to ADEP were recorded on an in-house SAXS instrument (SAXSess mc2, Anton Paar, Graz, Austria) equipped with a Kratky camera, a sealed X-ray tube source and a two-dimensional Princeton Instruments PI·SCX:4300 (Roper Scientific) CCD detector. The scattering patterns were measured with a 90-min exposure time (540 frames, each 10 s) for several solute concentrations in the range 1.8–8.2 mg ml −1 . Data for each sample was recorded at three different concentrations, that is, undiluted, at half concentration and one-fourth concentration. As no changes in the shape of the SAXS curves were observed for all samples recorded at different dilutions, the highest concentration with the best signal-to-noise ratio was selected to prepare the figures and for further analysis. Tag-free or C-terminal Strep-tagged proteins were purified by size exclusion chromatography prior to measurement. Samples were taken from the central peak fractions and treated with either ADEP4/7 (50 mM stocks in DMSO, final concentration range: 84–380 μM corresponding to a 1:1 ratio of ADEP:SaClpP) or the respective amount of DMSO (0.6% (v/v) max). Radiation damage was excluded based on a comparison of individual frames of the 90-min exposures, where no changes were detected. A range of momentum transfer of 0.012< s <0.63 Å −1 was covered ( s =4 π sin( θ )/ λ , where 2 θ is the scattering angle and λ =1.5 Å is the X-ray wavelength). All SAXS data were analyzed with the package ATSAS (version 2.5). The data were processed with the SAXSQuant software (version 3.9), and desmeared using the programmes GNOM [64] and GIFT [65] . The forward scattering, I (0), the radius of gyration, R g , the maximum dimension, D max , and the inter-atomic distance distribution functions, ( P ( R )), were computed with the programme GNOM. The masses of the solutes were evaluated by comparison of the forward scattering intensity with that of a human serum albumin reference solution (molecular mass 69 kDa). To generate ab initio shape models, a total number of 20 models were calculated using the programme DAMMIF [66] and aligned and averaged using the programme DAMAVER [67] . C72 and C7 symmetry was defined for tetradecameric and heptameric SaClpP, respectively. The ab initio shape models were aligned with crystal structures of SaClpP (PDB IDs 3V5E and 3QWD) using the programme SUPCOMB [68] . Dynamic light scattering Protein samples in buffer D (322 μM) with ADEP (322 μM) or DMSO (3%) were loaded into disposable plastic cuvettes. DLS was measured on a Wyatt DynaPro Nanostar laser photometer (662.3 nm) at 25 °C. For each sample, 10 measurements were performed, which consisted of 10 acquisitions each with an acquisition time of 5 s. Data were fit with Dynamics version 7 software to a multimodal spheric model. P values were calculated in OriginPro using an independent two-sample t -test ( N =10) with equal variances not assumed. SaClpXP assay Degradation assays were performed in PZ buffer (25 mM Hepes, 200 mM KCl, 5 mM MgCl 2 , 1 mM DTT, 10% (v/v) glycerol, pH 7.6) with 60 μl reaction volume at 30 °C. GFP fluorescence was monitored in white, flat-bottom well plates (Greiner) by exciting at 465 nm and measuring emission at 535 nm using an Infinite F200 Pro (Tecan). Degradation reactions contained 0.4 μM SaClpX 6 , 0.2 μM ClpP 14 , 0.36 μM GFP–ssrA and an ATP regeneration system (4 mM ATP, 16 mM creatine phosphate, 20 U ml −1 creatine phosphokinase). 0.6 μl (1% of reaction volume) ADEP was added in different concentrations in DMSO. All reaction partners except the substrate were pre-incubated for 10 min at 30 °C. GFP–ssrA was added to start the reaction. All data were recorded in triplicate measurements. GFP unfolding activity was derived as initial slopes in fluorescence time courses. Reactions were quenched after 3 h by addition of SDS sample buffer, and samples were analyzed both by denaturing and weakly denaturing SDS–PAGE for Coomassie and in-gel GFP fluorescence analysis, respectively. Binding site identification SaClpP (10 μM) was treated with β-lactone D3 (100 μM) in buffer D and incubated for 1 h at 25 °C. It was checked by protein mass spectrometry for complete modification and the sample was then buffer-exchanged to 50 mM ammonium bicarbonate (pH 7.3). Following a trypsin digest, peptides were analyzed on a LTQ Orbitrap XL mass spectrometer (Thermo Scientific) [39] . Data analysis was performed with the SEQUEST algorithm and the S. aureus NCTC 8325 proteome via Bioworks software allowing for covalent modification with D3 (monoisotopic mass: 262.1933, amu) on serine, threonine, cysteine, histidine and lysine residues. In vitro activity-based protein profiling SaClpP (1 μM) was incubated with alkyne-tagged β-lactones (50 μM) in buffer D for 1 h at room temperature in a total volume of 100 μl, and the entire procedure of click-chemistry-mediated attachment of a fluorophore, separation via SDS–PAGE and fluorescence scanning have been described previously [39] . See the Supplementary Methods and Supplementary Figs 8–12 for the synthesis of the four stereoisomers of β-lactone U1. How to cite this article: Gersch, M. et al. AAA+ chaperones and acyldepsipeptides activate the ClpP protease via conformational control. Nat. Commun. 6:6320 doi: 10.1038/ncomms7320 (2015).